Activation of the mitochondrial unfolded protein response does not predict longevity inCaenorhabditis elegans Recent studies have propagated the model that the mitochondrial unfolded protein response (UPR mt ) is causal for lifespan extension from inhibition of the electron transport chain (ETC) in Caenorhabditis elegans . Here we report a genome-wide RNAi screen for negative regulators of the UPR mt . Lifespan analysis of nineteen RNAi clones that induce the hsp-6 p ::gfp reporter demonstrate differential effects on longevity. Deletion of atfs-1 , which is required for induction of the UPR mt , fails to prevent lifespan extension from knockdown of two genes identified in our screen or following knockdown of the ETC gene cco-1 . RNAi knockdown of atfs-1 also has no effect on lifespan extension caused by mutation of the ETC gene isp-1 . Constitutive activation of the UPR mt by gain of function mutations in atfs-1 fails to extend lifespan. These observations identify several new factors that promote mitochondrial homoeostasis and demonstrate that the UPR mt , as currently defined, is neither necessary nor sufficient for lifespan extension. As the primary source of cellular energy and a major source of damage, mitochondria play an important role in modulating many age-related processes [1] , [2] . Harman first proposed the free radical theory of aging, which posits that damage resulting from reactive oxygen species (ROS) produced as a by-product of mitochondria metabolism determines the rate of organismal aging [3] . Recent studies have demonstrated that the situation is more complex than originally proposed, however, with important pro-longevity signalling functions of ROS having been established in several species [4] . The effect of mitochondria on aging has been studied thoroughly in the nematode Caenorhabditis elegans , where RNAi knockdown of several mitochondrial electron transport chain (ETC) genes has been shown to extend lifespan [5] , [6] . Knockdown of ETC genes must occur during a specific stage of development to promote longevity [7] , [8] , [9] , suggesting that a signal or altered metabolic state is established following ETC disruption during development to modulate adult longevity. The requirement of developmental disruption of ETC function to enhance longevity is distinct from most other longevity interventions, such as reduced insulin/IGF-1-like signalling or dietary restriction, which appear to act on aging primarily during adulthood [10] , [11] . The effect of ETC knockdown on lifespan is also dose-responsive, such that too much inhibition of ETC function during development can shorten lifespan [8] . A few mutations that impair mitochondrial function have also been shown to extend lifespan in C. elegans , including alleles of the coenzyme Q biosynthetic gene clk-1 (refs 12 , 13 ), the Rieske iron-sulphur protein gene isp-1 (ref. 14 ), and thiamine pyrophosphokinase gene tpk-1 (refs 15 , 16 ). Several factors have been suggested to directly promote lifespan extension from ETC knockdown and mitochondrial inhibition in C. elegans . For example, inhibition of ETC function can lead to increased levels of ROS, which can induce lifespan extension [17] , [18] . One effect of this ROS production is stabilization and activation of the hypoxia-inducible transcription factor HIF-1, which is also required for full lifespan extension in some mitochondrial mutants and RNAi knockdowns [18] . Stabilization of HIF-1 is sufficient to extend lifespan robustly through a mechanism that is also distinct from insulin/IGF-1-like signalling and dietary restriction [19] , [20] , [21] , [22] , providing a plausible explanation for lifespan extension in these cases. In addition to HIF-1, other factors have also been implicated in lifespan extension following inhibition of mitochondrial function. These include AMP-activated protein kinase [23] , the homeobox protein CEH-23 (ref. 24) [24] , the transcription factor TAF-4 (ref. 25) [25] and the p53 homologue CEP-1 (ref. 26) [26] . It remains unclear, however, whether any of these putative downstream mechanisms can account for a majority of the lifespan effects seen in the different long-lived models of mitochondrial inhibition. Recently, induction of the mitochondrial unfolded protein response (UPR mt ) was proposed to directly mediate lifespan extension from ETC inhibition in a cell non-autonomous manner [27] . The UPR mt is a stress response pathway first characterized in mammalian cells, whereby nuclear encoded mitochondrial chaperones are induced in response to misfolded proteins within the mitochondria or a stoichiometric imbalance of mitochondrial respiratory complexes [28] , [29] , [30] . The C. elegans UPR mt appears similar to that of mammals [27] , [31] , [32] , [33] , [34] , where induction of the UPR mt results in transcriptional upregulation of the mitochondrial chaperone genes hsp-6 and hsp-60 . RNAi knockdown of a subset of ETC components has been shown to induce the UPR mt in C. elegans using GFP reporters for both hsp-6 and hsp-60 (refs 27 , 31 ). In addition, the C. elegans UPR mt can only be induced robustly when mitochondrial stress precedes the L3/L4 larval stage transition [27] , a critical time period for mitochondrial biogenesis and longevity [8] , [35] . This signalling pathway is not completely understood, but several factors are reported to be required for full induction of the response, including the HAF-1 peptide exporter [34] , the CLPP-1 protease [33] , a ubiquitin-like protein UBL-5 (ref. 32) [32] and two transcription factors, DVE-1 and ATFS-1 (ZC376.7) [33] , [34] , [36] , [37] . Durieux et al. [27] linked the UPR mt to aging by showing that RNAi knockdown of UPR mt components can suppress the lifespan extension from mutations in isp-1 or clk-1 . Most of these knockdowns shortened the lifespan of wild-type animals, however, and also suppressed the lifespan extension associated with non-mitochondrial factors such as daf -2 and eat-2 , suggesting that the effects were non-specific. In one case, ubl-5(RNAi) , the suppression appeared to be specific for isp-1 and clk-1 , which was interpreted to indicate that induction of the UPR mt plays a causal role in lifespan extension from ETC inhibition [27] . This model was further supported by experiments showing that ubl-5(RNAi) can also partially or completely prevent lifespan extension from knockdown of cco-1 , which encodes cytochrome c oxidase subunit Vb/COX4, or mrps-5 , which encodes a mitochondrial ribosomal protein [38] . On the basis of the report by Durieux et al. [27] , we set out to identify additional genetic modifiers of lifespan by screening for RNAi clones that induce the UPR mt . Here we report the identification and validation of 25 previously unreported negative regulators of the UPR mt . Unexpectedly, several RNAi clones that induce the UPR mt shorten lifespan, and among at least a subset of those that extend lifespan, induction of the UPR mt is not required for lifespan extension. Constitutive activation of the UPR mt in the absence of mitochondrial stress also fails to extend lifespan. A genomic screen for negative regulators of the UPR mt We sought to identify RNAi clones that increase lifespan by screening for induction of fluorescence in animals expressing the hsp-6 p ::gfp reporter following RNAi knockdown of individual genes ( Fig. 1a ). 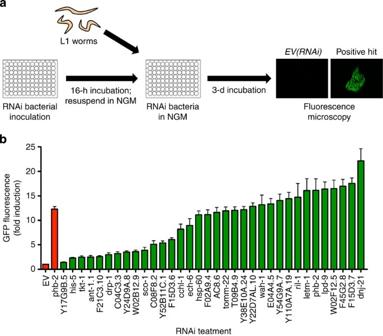Figure 1: A genome-wide RNAi screen for negative regulators of the mitochondrial unfolded protein response. (a) RNAi bacteria were grown overnight in 96-well plates, whilehsp-6p::gfpanimals were synchronized at L1 larval stage. The next day, RNAi bacteria was induced with IPTG, resuspended in liquid NGM and added to reporter animals in 96-well plates. Animals were allowed to develop for 3 days and GFP was measured by fluorescent microscopy. (b)hsp-6p::gfpinduction was quantified for 34 RNAi clones corresponding to positive hits that were not annotated as functioning in the ETC or mitochondrial translation. Validation included sequencing each RNAi clone and GFP quantification of individual animals grown at 20 °C. GFP fluorescence is the mean fluorescence relative toEV(RNAi)(N=3 independent experiments, error bars indicate s.e.m.). NGM, nematode growth media. We identified 95 putative inducers of the UPR mt from the Vidal ORFeome RNAi library (11,511 clones) ( Supplementary Table 1, 2 ). 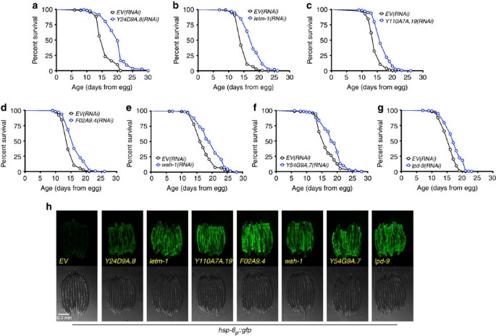Figure 2:Several UPRmt-inducing RNAi clones extend lifespan. (a) N2 fedEV(RNAi)(mean 15.8±0.2 days,n=284), N2 fedY24D9A.8(RNAi)(mean 19.8±0.2 days,n=316,P<0.0001). (b) N2 fedEV(RNAi)(mean 15.0±0.1 days,n=320), N2 fedletm-1(RNAi)(mean 18.1±0.2 days,n=318,P<0.0001). (c) N2 fedEV(RNAi)(mean 14.3±0.1 days,n=267), N2 fedY110A7A.19(RNAi)(mean 16.8±0.1 days,n=360,P<0.0001). (d) N2 fedEV(RNAi)(mean 14.6±0.1 days,n=266), N2 fedF02A9.4(RNAi)(mean 16.6±0.2 days,n=302,P<0.0001). (e) N2 fedEV(RNAi)(mean 17.4±0.2 days,n=264), N2 fedwah-1(RNAi)(mean 19.6±0.2 days,n=301,P<0.0001). (f) N2 fedEV(RNAi)(mean 16.5±0.2 days,n=279), N2 fedY54G9A.7(RNAi)(mean 18.5±0.2 days,n=266,P<0.0001). (g) N2 fedEV(RNAi)(mean 15.7±0.1 days,n=293), N2 fedlpd-9(RNAi)(mean 17.3±0.2 days,n=226,P<0.0001). (h) Thehsp-6p::gfpreporter is induced by knockdown of longevity conferring RNAi clones.hsp-6p::gfpworms were placed onto RNAi bacteria from egg and GFP measurements were taken 3 days later. Scale bar, 0.3 mm. Lifespan experiments in this figure were performed at 25 °C.n=3 independent experiments, with pooled data shown. Lifespan are indicated as mean±s.e.m. andP-values were calculated using Wilcoxon rank-sum test. Data by individual experiment and statistical analysis provided inSupplementary Materials(Supplementary Data 1). Of these, 39 RNAi clones target subunits of the ETC and 22 target mitochondrial ribosomal subunits or translation factors ( Supplementary Table 2 ). Of the 95 clones identified from this screen, 29 have been previously reported to induce the UPR mt [31] , [36] , [38] , [39] , [40] , [41] , and the remaining 66 are novel. Figure 1: A genome-wide RNAi screen for negative regulators of the mitochondrial unfolded protein response. ( a ) RNAi bacteria were grown overnight in 96-well plates, while hsp-6 p ::gfp animals were synchronized at L1 larval stage. The next day, RNAi bacteria was induced with IPTG, resuspended in liquid NGM and added to reporter animals in 96-well plates. Animals were allowed to develop for 3 days and GFP was measured by fluorescent microscopy. ( b ) hsp-6 p ::gfp induction was quantified for 34 RNAi clones corresponding to positive hits that were not annotated as functioning in the ETC or mitochondrial translation. Validation included sequencing each RNAi clone and GFP quantification of individual animals grown at 20 °C. GFP fluorescence is the mean fluorescence relative to EV(RNAi) ( N =3 independent experiments, error bars indicate s.e.m.). NGM, nematode growth media. Full size image Since ETC components and mitochondrial ribosomal proteins are known to modulate both the UPR mt and longevity [7] , [9] , [42] , we chose to further characterize RNAi clones identified from our screen that have not been shown to play a direct role in these processes. After sequence-validation of these RNAi clones, we focused on 34 that reproducibly induced expression of the hsp-6 p ::gfp reporter relative to empty vector RNAi ( Fig. 1b ). The targeted genes function in mitochondrial protein import, fat storage, sugar metabolism and other aspects of mitochondrial biology such as mitochondrial fission, protein quality control and ion transport ( Table 1 , Supplementary Table 1 ). Although several of the identified genes have not been shown to modulate mitochondrial function in C. elegans , some are homologous to known mitochondrial genes in other species or are expected to localize to the mitochondria on the basis of predicted mitochondrial targeting sequences ( Supplementary Table 1 ). 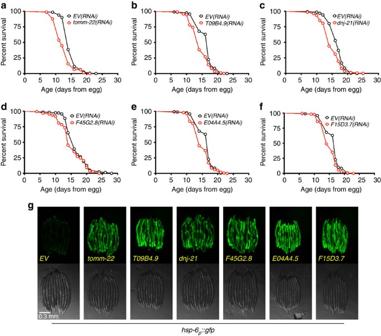Figure 3:Several UPRmt-inducing RNAi clones shorten lifespan. (a) N2 fedEV(RNAi) (mean 14.8±0.1 days,n=335), N2 fedtomm-22(RNAi)(mean 12.7±0.2 days,n=327,P<0.0001). (b) N2 fedEV(RNAi)(mean 16.3±0.2 days,n=260), N2 fedT09B4.9(RNAi)(mean 14.5±0.2 days,n=289,P<0.0001). (c) N2 fedEV(RNAi)(mean 16.7±0.1 days,n=293), N2 feddnj-21(RNAi)(mean 14.9±0.2 days,n=270,P<0.0001). (d) N2 fedEV(RNAi)(mean 16.5±0.2 days,n=279), N2 fedF45G2.8(RNAi)(mean 15.2±0.2 days,n=291,P<0.0001). (e) N2 fedEV(RNAi)(mean 16.3±0.2 days,n=260), N2 fedE04A4.5(RNAi)(mean 15.1±0.2 days,n=199,P<0.0001). (f) N2 fedEV(RNAi)(mean 16.3±0.2 days,n=260), N2 fedF15D3.7(RNAi)(mean 15.1±0.2 days,n=217,P<0.0001). (g) Thehsp-6p::gfpreporter is induced by knockdown of RNAi clones that reduce lifespan.hsp-6p::gfpworms were placed onto RNAi bacteria from egg and grown at 25 °C. GFP measurements were taken 3 days later. Scale bar, 0.3 mm. Lifespan experiments in this figure were performed at 25 °C.n=3 independent experiments, with pooled data shown. Lifespans are indicated as mean±s.e.m. andP-values were calculated using Wilcoxon rank-sum test. Data by individual experiment and statistical analysis provided inSupplementary Materials(Supplementary Data 1). About half (18/34) of the RNAi clones that induced expression of the hsp-6 p ::gfp reporter also significantly induced expression of the mitochondrial hsp-60 p ::gfp reporter, while none of the RNAi clones induced reporters of either the endoplasmic reticulum UPR ( hsp-4 p ::gfp ) or the cytoplasmic heat shock response ( hsp-16.2 p ::gfp ) to a detectable level, with the exception of Y38E10A.24 ( RNAi ), which modestly increased fluorescence in the hsp-4 p ::gfp strain ( Supplementary Table 3 ). Table 1 Effects of 19 UPR mt regulators on lifespan. Full size table Relationship between the UPR mt and longevity On the basis of the model that lifespan extension from ETC inhibition results from induction of the UPR mt , we predicted that a majority of the clones identified from our screen would extend lifespan. Out of 19 RNAi clones tested, ten significantly increased lifespan ( P <0.05, Wilcoxon rank-sum, Table 1 ), of which seven increased lifespan by more than ten percent ( Fig. 2a–g ). Six other RNAi clones significantly decreased mean lifespan ( Fig. 3a–f ). No correlation between UPR mt induction and lifespan was detected for knockdowns that significantly affected lifespan ( Figs 2h , 3g and 4 ). Notably, all of the clones that significantly reduced lifespan correspond to worm homologues of proteins important for transport of mitochondrial-localized proteins into the mitochondria. These included tomm-22 , a component of the TOM complex which functions as a translocase in the outer mitochondrial membrane and E04A4.5 (TIM17), T09B4.9 (TIM44), F45G2.8 (TIM16), F15D3.7 (TIM23), and dnj-21 (TIM14), which function in the TIM23 complex that transports proteins into the inner membrane and the matrix [43] , [44] . The RNAi clones that significantly increased lifespan appear to correspond to functionally diverse proteins. These include LETM-1, a mitochondrial transmembrane protein involved in potassium homoeostasis that is associated with seizures in Wolf–Hirschhorn syndrome patients, LPD-9, a protein involved in fat storage, and Y24D9A.8 , which is orthologous to human TALDO1 encoding transaldolase, an enzyme of the pentose phosphate pathway. Figure 2: Several UPR mt -inducing RNAi clones extend lifespan. ( a ) N2 fed EV(RNAi) (mean 15.8±0.2 days, n =284), N2 fed Y24D9A.8(RNAi) (mean 19.8±0.2 days, n =316, P <0.0001). ( b ) N2 fed EV(RNAi) (mean 15.0±0.1 days, n =320), N2 fed letm-1(RNAi) (mean 18.1±0.2 days, n =318, P <0.0001). ( c ) N2 fed EV(RNAi) (mean 14.3±0.1 days, n =267), N2 fed Y110A7A.19(RNAi) (mean 16.8±0.1 days, n =360, P <0.0001). ( d ) N2 fed EV(RNAi) (mean 14.6±0.1 days, n =266), N2 fed F02A9.4(RNAi) (mean 16.6±0.2 days, n =302, P <0.0001). ( e ) N2 fed EV(RNAi) (mean 17.4±0.2 days, n =264), N2 fed wah-1(RNAi) (mean 19.6±0.2 days, n =301, P <0.0001). ( f ) N2 fed EV(RNAi) (mean 16.5±0.2 days, n =279), N2 fed Y54G9A.7(RNAi) (mean 18.5±0.2 days, n =266, P <0.0001). ( g ) N2 fed EV(RNAi) (mean 15.7±0.1 days, n =293), N2 fed lpd-9(RNAi) (mean 17.3±0.2 days, n =226, P <0.0001). ( h ) The hsp-6 p ::gfp reporter is induced by knockdown of longevity conferring RNAi clones. hsp-6 p ::gfp worms were placed onto RNAi bacteria from egg and GFP measurements were taken 3 days later. Scale bar, 0.3 mm. Lifespan experiments in this figure were performed at 25 °C. n =3 independent experiments, with pooled data shown. Lifespan are indicated as mean±s.e.m. and P -values were calculated using Wilcoxon rank-sum test. Data by individual experiment and statistical analysis provided in Supplementary Materials ( Supplementary Data 1 ). Full size image Figure 3: Several UPR mt -inducing RNAi clones shorten lifespan. ( a ) N2 fed EV(RNAi) ( mean 14.8±0.1 days, n =335), N2 fed tomm-22(RNAi) (mean 12.7±0.2 days, n =327, P <0.0001). ( b ) N2 fed EV(RNAi) (mean 16.3±0.2 days, n =260), N2 fed T09B4.9(RNAi) (mean 14.5±0.2 days, n =289, P <0.0001). ( c ) N2 fed EV(RNAi) (mean 16.7±0.1 days, n =293), N2 fed dnj-21(RNAi) (mean 14.9±0.2 days, n =270, P <0.0001). ( d ) N2 fed EV(RNAi) (mean 16.5±0.2 days, n =279), N2 fed F45G2.8(RNAi) (mean 15.2±0.2 days, n =291, P <0.0001). ( e ) N2 fed EV(RNAi) (mean 16.3±0.2 days, n =260), N2 fed E04A4.5(RNAi) (mean 15.1±0.2 days, n =199, P <0.0001). ( f ) N2 fed EV(RNAi) (mean 16.3±0.2 days, n =260), N2 fed F15D3.7(RNAi) (mean 15.1±0.2 days, n =217, P <0.0001). ( g ) The hsp-6 p ::gfp reporter is induced by knockdown of RNAi clones that reduce lifespan. hsp-6 p ::gfp worms were placed onto RNAi bacteria from egg and grown at 25 °C. GFP measurements were taken 3 days later. Scale bar, 0.3 mm. Lifespan experiments in this figure were performed at 25 °C. n =3 independent experiments, with pooled data shown. Lifespans are indicated as mean±s.e.m. and P -values were calculated using Wilcoxon rank-sum test. Data by individual experiment and statistical analysis provided in Supplementary Materials ( Supplementary Data 1 ). 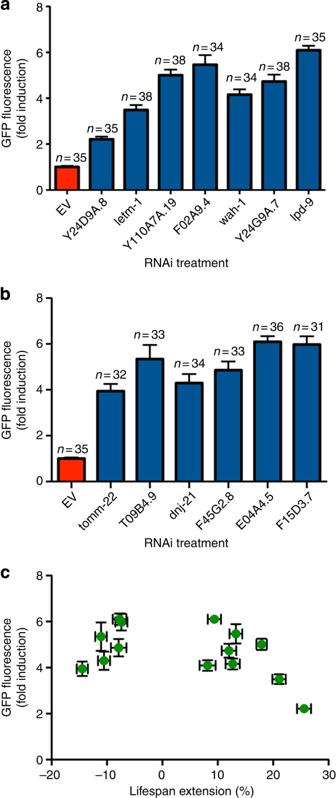Figure 4:Induction ofhsp-6p::gfpis not correlated with lifespan extension. hsp-6p::gfpinduction from three separate experiments performed at 25 °C for (a) long-lived RNAi clones and (b) short-lived RNAi clones. GFP fluorescence is the average fluorescence of an individual worm relative toEV(RNAi)and error bars indicate s.e.m. (c)hsp-6p::gfpinduction is not significantly positively correlated with lifespan extension. The Pearson’s correlationR2is 0.1912 andP-value is 0.12. Error bars indicate s.e.m. for GFP fluorescence and % mean lifespan extension relative toEV(RNAi). Full size image Figure 4: Induction of hsp-6 p ::gfp is not correlated with lifespan extension. hsp-6 p ::gfp induction from three separate experiments performed at 25 °C for ( a ) long-lived RNAi clones and ( b ) short-lived RNAi clones. GFP fluorescence is the average fluorescence of an individual worm relative to EV(RNAi) and error bars indicate s.e.m. ( c ) hsp-6 p ::gfp induction is not significantly positively correlated with lifespan extension. The Pearson’s correlation R 2 is 0.1912 and P -value is 0.12. Error bars indicate s.e.m. for GFP fluorescence and % mean lifespan extension relative to EV(RNAi) . Full size image ATFS-1 is required for UPR mt induction but not longevity We next set out to more directly characterize the role of the UPR mt in lifespan extension from knockdown of two of the novel longevity clones identified from our screen: letm-1 and Y24D9A.8 (transaldolase). We first considered using the haf-1(ok705) mutant for epistasis experiments, but found that haf-1 was not required for induction of the UPR mt caused by RNAi knockdown of cco-1 or by RNAi knockdown of the gene encoding the mitochondrial prohibitin phb-2 ( Supplementary Fig. 1 ). Therefore, we utilized the atfs-1(tm4525) mutation, which has been shown to prevent induction of the UPR mt following knockdown of mitochondrial AAA-protease spg-7 , knockdown of mitochondrial import machinery, and ethidium bromide treatment [36] . In the absence of mitochondrial stress, ATFS-1 is imported into the mitochondria where it is degraded; when mitochondria are dysfunctional, import and degradation of ATFS-1 is impaired and it relocalizes to the nucleus to induce expression of UPR mt genes, including hsp-6 and hsp-60 (ref. 36 ). On the basis of the model that the UPR mt plays a causal role in lifespan extension, we reasoned that RNAi of either letm-1 or Y24D9A.8 (transaldolase) should have no effect on lifespan in the atfs-1(tm4525) background. Unexpectedly, deletion of atfs-1 failed to significantly attenuate the lifespan extension from RNAi knockdown in either case ( Fig. 5a,b ). 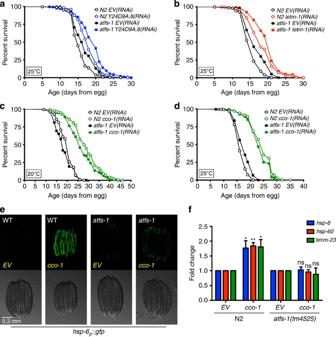Figure 5:UPRmt-inducing RNAi clones do not requireatfs-1for lifespan extension. (a)Y24D9A.8(RNAi)lifespan extension is not dependent onatfs-1. N2 fedEV(RNAi)(mean 15.7±0.1 days,n=535), N2 fedY24D9A.8(RNAi)(mean 18.1±0.1 days,n=456,P<0.0001),atfs-1(tm425)fedEV(RNAi)(mean 17±0.2 days,n=417),atfs-1(tm4525)fedY24D9A.8(RNAi)(19.2±0.2 days,n=334,P<0.0001). (b)letm-1(RNAi)lifespan extension is not dependent onatfs-1. N2 fedEV(RNAi)(mean 15.5±0.1,n=460), N2 fedletm-1(RNAi)(mean 18.6±0.2,n=421,P<0.0001),atfs-1(tm425)fedEV(RNAi)(mean 17±0.2,n=386),atfs-1(tm4525)fedletm-1(RNAi)(mean 20.1±0.2,n=358,P<0.0001). (c) The long lifespan ofcco-1(RNAi)is not dependent onatfs-1at 20 °C. N2 fedEV(RNAi)(mean 19.9±0.2,n=215), N2 fedcco-1(RNAi)(mean 28.9±0.5,n=170,P<0.0001),atfs-1(tm425)fedEV(RNAi)(mean 18.6±0.3,n=202),atfs-1(tm4525)fedcco-1(RNAi)(mean 26.9±0.5,n=170,P<0.0001). (d) The long lifespan ofcco-1(RNAi)is not dependent onatfs-1at 25 °C. N2 fedEV(RNAi)(mean 16.6±0.1,n=279), N2 fedcco-1(RNAi)(mean 24.2±0.3,n=242,P<0.0001),atfs-1(tm425)fedEV(RNAi)(mean 17.8±0.2,n=302),atfs-1(tm4525)fedcco-1(RNAi)(mean 23.5±0.3,n=202,P<0.0001). (e)hsp-6p::gfpinduction bycco-1(RNAi)is attenuated in theatfs-1(tm4525)mutant. Scale bar, 0.3 mm. (f) Induction of UPRmttargetshsp-6,hsp-60, andtimm-23does not occur in theatfs-1(tm4525)mutant. N2 andatfs-1(tm4525)worms were grown oncco-1(RNAi)from egg at 20 °C and harvested at L4. Gene expression was normalized toEV(RNAi). (n=4, Error bars represent s.e.m., *P<0.05, **P<0.01),P>0.05 is not significant (NS), student’st-test). Lifespan experiments in this figure represent pooled data, are indicated as mean±s.e.m., andP-values were calculated using Wilcoxon rank-sum test. Data by individual experiment and statistical analysis provided inSupplementary Materials(Supplementary Data 2). WT, wild type. Figure 5: UPR mt -inducing RNAi clones do not require atfs-1 for lifespan extension. ( a ) Y24D9A.8(RNAi) lifespan extension is not dependent on atfs-1 . N2 fed EV(RNAi) (mean 15.7±0.1 days, n =535), N2 fed Y24D9A.8(RNAi) (mean 18.1±0.1 days, n =456, P <0.0001), atfs-1(tm425) fed EV(RNAi) (mean 17±0.2 days, n =417), atfs-1(tm4525) fed Y24D9A.8(RNAi) (19.2±0.2 days, n =334, P <0.0001). ( b ) letm-1(RNAi) lifespan extension is not dependent on atfs-1 . N2 fed EV(RNAi) (mean 15.5±0.1, n =460), N2 fed letm-1(RNAi) (mean 18.6±0.2, n =421, P <0.0001), atfs-1(tm425) fed EV(RNAi) (mean 17±0.2, n =386), atfs-1(tm4525) fed letm-1(RNAi) (mean 20.1±0.2, n =358, P <0.0001). ( c ) The long lifespan of cco-1(RNAi) is not dependent on atfs-1 at 20 °C. N2 fed EV(RNAi) (mean 19.9±0.2, n =215), N2 fed cco-1(RNAi) (mean 28.9±0.5, n =170, P <0.0001), atfs-1(tm425) fed EV(RNAi) (mean 18.6±0.3, n =202), atfs-1(tm4525) fed cco-1(RNAi) (mean 26.9±0.5, n =170, P <0.0001). ( d ) The long lifespan of cco-1(RNAi) is not dependent on atfs-1 at 25 °C. N2 fed EV(RNAi) (mean 16.6±0.1, n =279), N2 fed cco-1(RNAi) (mean 24.2±0.3, n =242, P <0.0001), atfs-1(tm425) fed EV(RNAi) (mean 17.8±0.2, n =302), atfs-1(tm4525) fed cco-1(RNAi) (mean 23.5±0.3, n =202, P <0.0001). ( e ) hsp-6 p ::gfp induction by cco-1(RNAi) is attenuated in the atfs-1(tm4525) mutant. Scale bar, 0.3 mm. ( f ) Induction of UPR mt targets hsp-6 , hsp-60 , and timm-23 does not occur in the atfs-1(tm4525) mutant. N2 and atfs-1(tm4525) worms were grown on cco-1(RNAi) from egg at 20 °C and harvested at L4. Gene expression was normalized to EV(RNAi) . ( n =4, Error bars represent s.e.m., * P <0.05, ** P <0.01), P >0.05 is not significant (NS), student’s t -test). Lifespan experiments in this figure represent pooled data, are indicated as mean±s.e.m., and P -values were calculated using Wilcoxon rank-sum test. Data by individual experiment and statistical analysis provided in Supplementary Materials ( Supplementary Data 2 ). WT, wild type. Full size image To determine whether the lack of effect from atfs-1 deletion on lifespan extension is specific to these newly identified UPR mt -inducing clones, we asked whether knockdown of cco-1 , which is already known to extend lifespan [7] , [8] , [9] , was dependent on atfs-1 . To rule out the possibility that high temperature (25 °C) could influence the outcome by modulating expression of UPR mt genes independently of the mitochondrial stress, we performed subsequent experiments at 20 °C in addition to 25 °C. Once again, deletion of atfs-1 failed to significantly attenuate lifespan extension from cco-1(RNAi) at both temperatures ( Fig. 5c,d ). The presence of the atfs-1(tm4525) allele was verified by PCR ( Supplementary Fig. 2 ), and deletion of atfs-1 prevented induction of both hsp-6 p ::gfp reporter, as well as three different endogenous UPR mt genes, hsp-6 , hsp-60 and timm-23 , following cco-1(RNAi) ( Fig. 5e,f ). To further test the generality of our observations, we treated long-lived isp-1(qm150) mutant animals with atfs-1(RNAi) . As has been previously reported [36] , we confirmed that atfs-1(RNAi) delayed the development of isp-1 mutant animals ( Supplementary Fig. 3 ). Even when this delay is taken into account, mutation of isp-1 significantly increased the lifespan of animals treated with atfs-1(RNAi) comparably to animals treated with empty vector RNAi ( Fig. 6a ), despite the fact that atfs-1(RNAi) completely prevented induction of GFP in isp-1(qm150) animals expressing the hsp-6 p ::gfp reporter ( Fig. 6b ). 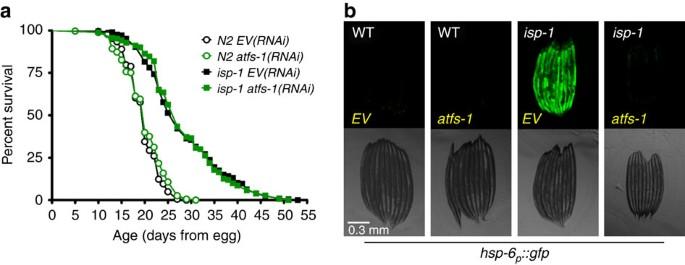Figure 6:The UPRmtis not required forisp-1(qm150)longevity. (a) Knockdown ofatfs-1does not attenuate the longevity of complex III mutantisp-1(qm150). N2 fedEV(RNAi)(mean 19.7±0.2,n=365), N2 fedatfs-1(RNAi)(mean 20±0.2 days,n=346,P=0.399),isp-1(qm150)fedEV(RNAi)(mean 28.2±0.6 days,n=206),isp-1(qm150)fedatfs-1(RNAi)(mean 28.3±0.5 days,n=293,P=0.612). (b)hsp-6p::gfpinduction byisp-1(qm150)mutation is attenuated byatfs-1(RNAi). Scale bar, 0.3 mm. Lifespan experiments in this figure represent pooled data, are indicated as mean±s.e.m., andP-values were calculated using Wilcoxon rank-sum test. Data by individual experiment and statistical analysis provided inSupplementary Materials(Supplementary Data 2). WT, wild type. Figure 6: The UPR mt is not required for isp-1(qm150) longevity. ( a ) Knockdown of atfs-1 does not attenuate the longevity of complex III mutant isp-1(qm150) . N2 fed EV(RNAi) (mean 19.7±0.2, n =365), N2 fed atfs-1(RNAi) (mean 20±0.2 days, n =346, P =0.399), isp-1(qm150) fed EV(RNAi) (mean 28.2±0.6 days, n =206), isp-1(qm150) fed atfs-1(RNAi) (mean 28.3±0.5 days, n =293, P =0.612). ( b ) hsp-6 p ::gfp induction by isp-1(qm150) mutation is attenuated by atfs-1(RNAi) . Scale bar, 0.3 mm. Lifespan experiments in this figure represent pooled data, are indicated as mean±s.e.m., and P -values were calculated using Wilcoxon rank-sum test. Data by individual experiment and statistical analysis provided in Supplementary Materials ( Supplementary Data 2 ). WT, wild type. Full size image Stabilization of ATFS-1 does not extend lifespan Recently, constitutively active alleles of ATFS-1 have been described which result in induction of the UPR mt in the absence of exogenous mitochondrial stress [45] . To determine whether constitutive activation of the UPR mt is sufficient to extend lifespan in the absence of ETC inhibition, we measured the lifespans of strains carrying either the atfs-1(et17) or atfs-1(et18) alleles. In both cases, lifespan was significantly reduced at 20 °C, rather than extended ( Fig. 7a,b ). Similar results were obtained at 25 °C, although the reduction in lifespan was attenuated at the higher temperature ( Fig. 7c,d ). The endogenous UPR mt targets hsp-6 , hsp-60 and timm-23 were significantly induced in the atfs-1(et17) and atfs-1(et18) strains, relative to N2 ( Fig. 7e ), demonstrating constitutive activation of the UPR mt in these animals. 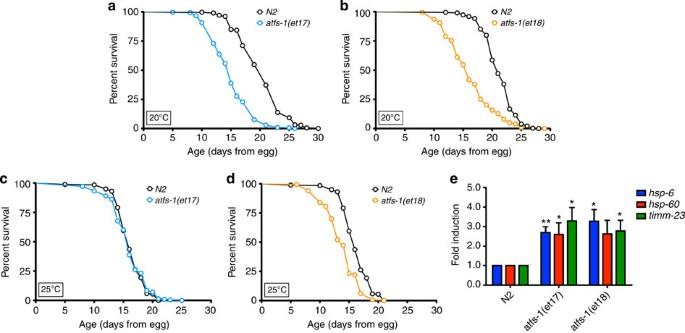Figure 7:The UPRmtis not sufficient for lifespan extension. (a) Constitutive UPRmtmutationatfs-1(et17)shortens lifespan at 20 °C. N2 fed HT115 bacteria (mean 20.3±0.2 days,n=312),atfs-1(et17)fed HT115 bacteria (mean 15±0.2,n=303,P<0.0001). (b) Constitutive UPRmtmutationatfs-1(et18)shortens lifespan at 20 °C. N2 fed HT115 bacteria (mean 21.3±0.1,n=418),atfs-1(et18)fed HT115 bacteria (mean 16.3±0.3 days,n=203,P<0.0001). (c)atfs-1(et17)mutation does not affect lifespan at 25 °C. N2 fed HT115 bacteria (mean=16.2±0.15 days),atfs-1(et17)fed HT115 bacteria (mean=15.9±0.21 days,P=0.31). (d)atfs-1(et18)mutation shortens lifespan at 25 °C. N2 fed HT115 bacteria (mean=16.2±0.15 days),atfs-1(et18)fed HT115 bacteria (mean=13.8±0.13 days,P<0.0001). (e) Constitutive UPRmtmutationsatfs-1(et17)andatfs-1(et18)induce expression ofhsp-6,hsp-60, andtimm-23. Gene expression was normalized to N2 fedEV(RNAi). (n=4, Error bars represent s.e.m., *P<0.05, **P<0.01, student’st-test). The gene expression data forhsp-60in theatfs-1(et18) alleleis trending significant, withP=0.05. Lifespan experiments in this figure represent pooled data, are indicated as mean±s.e.m., andP-values were calculated using Wilcoxon rank-sum test. Data by individual experiment and statistical analysis provided inSupplementary Materials(Supplementary Data 2). Figure 7: The UPR mt is not sufficient for lifespan extension. ( a ) Constitutive UPR mt mutation atfs-1(et17) shortens lifespan at 20 °C. N2 fed HT115 bacteria (mean 20.3±0.2 days, n =312), atfs-1(et17) fed HT115 bacteria (mean 15±0.2, n =303, P <0.0001). ( b ) Constitutive UPR mt mutation atfs-1(et18) shortens lifespan at 20 °C. N2 fed HT115 bacteria (mean 21.3±0.1, n =418), atfs-1(et18) fed HT115 bacteria (mean 16.3±0.3 days, n =203, P <0.0001). ( c ) atfs-1(et17) mutation does not affect lifespan at 25 °C. N2 fed HT115 bacteria (mea n =16.2±0.15 days), atfs-1(et17) fed HT115 bacteria (mea n =15.9±0.21 days, P =0.31). ( d ) atfs-1(et18) mutation shortens lifespan at 25 °C. N2 fed HT115 bacteria (mea n =16.2±0.15 days), atfs-1(et18) fed HT115 bacteria (mea n =13.8±0.13 days, P <0.0001). ( e ) Constitutive UPR mt mutations atfs-1(et17) and atfs-1(et18) induce expression of hsp-6 , hsp-60 , and timm-23 . Gene expression was normalized to N2 fed EV(RNAi) . ( n =4, Error bars represent s.e.m., * P <0.05, ** P <0.01, student’s t -test). The gene expression data for hsp-60 in the atfs-1 ( et18) allele is trending significant, with P =0.05. Lifespan experiments in this figure represent pooled data, are indicated as mean±s.e.m., and P -values were calculated using Wilcoxon rank-sum test. Data by individual experiment and statistical analysis provided in Supplementary Materials ( Supplementary Data 2 ). Full size image The model that the UPR mt plays a causal role in lifespan extension has become widely accepted, despite the correlative nature of the supporting data and the lack of evidence that induction of the UPR mt is sufficient to increase lifespan. In this study, we identified 95 gene knockdowns that induce the UPR mt , 66 of which are novel, and found that, at least for the subset tested here, there was no correlation between lifespan extension and the degree of UPR mt induction. Furthermore, we found that the UPR mt is neither necessary nor sufficient for lifespan extension by utilizing both null and gain of function mutations in the UPR mt transcription factor ATFS-1. As with prior studies of mitochondrial function in C. elegans , the studies described here are limited to mutations and RNAi knockdowns that only partially impair ETC function, since complete absence of ETC function is incompatible with life. Thus, we anticipate that additional genetic modifiers of the UPR mt , which may have resulted in lethality or early larval arrest in our RNAi screen, remain to be identified. This is consistent with prior studies indicating that RNAi knockdown of some mitochondrial factors results in severe lifespan reduction or lethality when the RNAi is undiluted, but increase lifespan when the RNAi is diluted or initiated post-developmentally [8] , [26] , [42] . The best evidence that the UPR mt directly promotes longevity comes from epistasis experiments reporting that knockdown of ubl-5 or haf-1 , which are required for full induction of the UPR mt , prevents lifespan extension from isp-1(qm150) or RNAi knockdown of either cco-1 or mrps-5 (refs 27 , 38 ). One major caveat to these experiments, however, is that neither ubl-5(RNAi) nor haf-1(RNAi) actually prevented induction of the UPR mt in these experiments. For example, in the study from Houtkooper et al. [38] , double knockdown of mrps-5 and haf-1 still resulted in an approximately 15-fold induction of the hsp-6 p ::gfp reporter relative to control animals, suggesting that the UPR mt is, at best, attenuated. Furthermore, no analysis of endogenous expression UPR mt targets was reported in these studies. In addition, we found that haf-1 is not required for induction of the UPR mt caused by knockdown of two additional mitochondrial genes: cco-1 and phb-2 . In the case of ubl- 5, which encodes an ubiquitin-like peptide homologous to the yeast splicing factor Hub1 (ref. 46) [46] , interpretation is further complicated by the fact that this protein likely has numerous functions beyond modulating the UPR mt . For these reasons, we felt that loss of atfs-1 , which has no known function outside of the UPR mt , might provide a useful alternative test of this model. In contrast to knockdown of either haf-1 or ubl-5 , we were able to demonstrate that deletion or RNAi knockdown of atfs-1 largely or completely abolishes induction of both the hsp-6 p ::gfp reporter and endogenous expression of three different UPR mt components ( hsp-6 , hsp-60 and timm-23 ), while having minimal effect on lifespan extension from multiple forms of mitochondrial stress, including mutation of isp-1 , RNAi knockdown of cco-1 and RNAi knockdown of two new aging genes identified in this study: letm-1 and Y24D9A.8 . Our observations that longevity is reduced by constitutive activation of ATFS-1 or by a subset of RNAi clones related to mitochondrial protein import ( tomm-22 , E04A4.5 , T09B4.9 , F45G2.8 , F15D3.7 and dnj-21 ), further argue against a direct causal link between the UPR mt and longevity, and demonstrate that activation of the UPR mt is not sufficient to enhance longevity. This is also consistent with prior reports showing that knockdown of the gene encoding the mitochondrial prohibitin phb-2 induces the UPR mt in both yeast and worms while simultaneously shortening lifespan in both organisms [47] , [48] . In the case of prohibitin deficiency, the lifespan defects can be suppressed by a reduction in cytoplasmic translation in yeast or by deletion of the S6 kinase homologue rsks-1 in worms, which both attenuate the UPR mt . It will be of interest to determine whether loss of rsks-1 or deletion of atfs-1 can prevent lifespan shortening in response to knockdown of mitochondrial protein import machinery. Although we reach a different conclusion with respect to the role of the UPR mt in longevity than has been previously suggested, the data presented in this study are generally consistent with the prior data from Durieux et al. [27] and Houtkooper et al. [38] . Our data also do not address the “mitokine” mechanism proposed by Durieux et al. [27] , whereby a neuronal signal is transmitted to distal cells to induce the UPR mt in a cell non-autonomous manner. By utilizing both RNAi and mutant alleles of atfs-1 , however, we are able to exclude the possibility that the presence (or absence) of neuronal UPR mt signalling (knockdown by RNAi feeding is generally less efficient in neurons) could yield different outcomes with respect to lifespan. It is also important to consider that the UPR mt is still relatively poorly characterized and imprecisely defined. Nearly every study of the UPR mt in C. elegans has utilized either the hsp-6 p ::gfp reporter or the hsp-60 p ::gfp reporter, with analysis of endogenous expression of hsp-6 , hsp-60 or other UPR mt targets rarely performed. Our data indicate that some RNAi clones that robustly induce expression of hsp-6 p ::gfp do not strongly induce expression of hsp-60 p ::gfp ( Supplementary Table 3 ). Whether this represents a biologically relevant difference in regulation of hsp-6 and hsp-60 or simply reflects differential sensitivities of the two reporters will require further study, but it does point out the possibility that there may be substantial differences in regulation of individual UPR mt targets, depending on the type of mitochondrial stress and the resulting signals from the mitochondria to the nucleus. For this reason, we chose to directly quantify mRNA levels for three UPR mt -regulated genes, in addition to utilizing these GFP reporter strains. In each case, similar changes in expression were observed. Our data therefore dissociate the UPR mt , as commonly defined in the field, from longevity; however, it remains possible that additional, as yet unknown, UPR mt targets that are regulated independently of ATFS-1 could influence lifespan directly. Thus, although we do not completely rule out a causal role for the UPR mt in aging, our data strongly suggest that if the UPR mt does play any direct longevity-promoting role. it is subtle, variable and highly context-dependent. Indeed, our interpretation of the entire body of data is that a stronger case can be made that the UPR mt generally suppresses longevity, and that inhibition of ETC function increases lifespan in spite of, rather than because of, the UPR mt . Our observation that the lifespan-extending RNAi clones, which also induce the UPR mt appear to encompass a range of mitochondrial and cytoplasmic functions suggests that the mechanisms by which mitochondrial perturbations modulate aging in C. elegans may extend beyond reduced ETC function or inhibition of mitochondrial translation. The fact that each of these RNAi clones also induces the UPR mt indicates that they are likely perturbing mitochondrial homoeostasis, or at least inducing a signal of mitochondrial stress. It will be important to understand how each of these factors is influencing mitochondrial function, particularly in those cases where there is no obvious link to mitochondria, such as transaldolase deficiency. In this regard, it is interesting to note that altered expression of pentose phosphate pathway enzymes has been associated with lifespan extension from calorie restriction in rhesus monkeys [49] , and transaldolase deficiency in mice causes loss of mitochondrial membrane potential and morphology in spermatozoa [50] . In addition to the UPR mt , several cellular pathways and factors have been proposed to mediate enhanced longevity following mitochondrial stress in C. elegans . As with prior studies on the UPR mt , however, each of these factors (for example, HIF-1, CEH-23, AMP kinase, p53/cep-1, TAF-4) have only been tested relative to one or a few long-lived mutants or RNAi clones. For now, it remains an open question as to whether a single mechanism will ultimately explain all of the various mitochondrial longevity interventions, or if multiple overlapping but distinct mechanisms contribute. Given the central role of mitochondrial function in metabolism, nutrient response and energetics, it is perhaps not surprising that the role of mitochondria in aging is complex and challenging to understand solely through genetic analyses. Taken together with prior studies, the observations reported here demonstrate that the relationship between the UPR mt and aging is significantly more complex than currently appreciated. At best, induction of the UPR mt is only weakly correlated with longevity, since many RNAi clones that induce the UPR mt either have no effect on lifespan or reduce lifespan, and induction of the UPR mt in the absence of mitochondrial stress fails to increase lifespan. Of the additional factors previously implicated in mitochondrial longevity, it remains unclear whether any represent a unifying mechanism. Despite the mechanistic uncertainties, however, the identification here of several novel RNAi clones that induce the UPR mt , at least eight of which also extend lifespan, further emphasizes the central importance of this pathway and suggests that this will be a fertile area for future research and insights into the fundamental mechanisms of mitochondrial quality control and aging. Strains NQ887 (isp-1(qm150)) , QC117 ( atfs-1(et17) ), QC118 ( atfs-1(et18) ), SJ4100 (zcIs13[ hsp-6 p ::gfp ]), SJ4058 (zcIs9[ hsp-60 p ::gfp ]), CL2070 (dvIs[ hsp-16.2 p ::gfp ]) and SJ4005 (zcIs4[ hsp-4 p ::gfp ]) were obtained from the Caenorhabditis Genetics Centre (Minneapolis, MN, USA). The atfs-1(tm4525) was obtained from the National BioResource Project (Tokyo, Japan) and backcrossed to our lab N2 strain twice. RNAi Screen and fluorescence microscopy All fluorescence microscopy was performed using a Zeiss SteREO Lumar.V12 microscope (Thornwood, NY, USA). The RNAi screen was performed using the Vidal RNAi library [51] and hsp-6 p ::gfp worms. RNAi bacteria were inoculated into LB Amp media and GFP reporter worms were hypochlorite treated and hatched in M9 overnight. The next day, RNAi bacteria were induced with 4 mM isopropyl-β-D-thiogalactoside (IPTG) for 1 hour, pelleted and resuspended in liquid nematode growth media supplemented with ampicillin and IPTG. RNAi bacteria were then added to 96-well plates with ~30 L1 reporter worms per well. After 3 days, GFP fluorescence was assessed manually by scoring photos as weak induction, strong induction or no induction. For validation of RNAi clones and quantification of different GFP reporter expression, GFP fluorescence of individual worms was quantified using IMAGEJ (Rasband, 1997–2012). Relative fluorescence to empty vector was calculated and fluorescence data were pooled across three independent experiments. A Student’s t -test was used to calculate significance with a Bonferonni correction to account for multiple comparisons. Synchronized eggs were grown on RNAi bacteria at 20 °C, unless otherwise stated. After 3 days, worms were assayed for GFP expression by fluorescence microscopy. For the hsp-16.2 p ::gfp and hsp-4 p ::gfp reporters, expression was induced by treatment with 4+ hour 30 °C heat shock and tunicamycin, respectively. At least two independent experiments, with approximately 10 animals per condition per experiment, performed on different days from different RNAi cultures, was obtained for each reporter with similar results. Lifespan analyses Lifespans were performed as described previously [52] . Synchronized eggs obtained by treating adult animals with hypochlorite were grown on nematode growth media plates containing 4 mM IPTG, 25 μg ml −1 carbenicillin and seeded with HT115(DE3) RNAi bacteria. At larval stage 4, worms were transferred to plates with 50 μM 5-fluoro-2′-deoxyuridine to prevent hatching of progeny. Lifespans were performed at 25 °C for the lifespan screen and at 20 °C and 25 °C in other experiments as described in the text and figures. Cohorts were examined every 1–3 days using tactile stimulation to verify viability of animals. Animals lost due to foraging were not included in the analysis. All lifespan analyses were replicated using independent cohorts on different dates with replicate statistics provided in Supplementary Materials ( Supplementary Data 1, 2 ). P -values were calculated using the Wilcoxon rank-sum test. GraphPad Prism was used for Pearson’s correlation statistics of hsp-6 p ::gfp induction versus lifespan. Quantitative RT–PCR RNA was isolated from L4 worms using a TRIzol (Life Technologies) chloroform extraction and cDNA was prepared according to the SuperScript III First Strand Synthesis protocol (Life Technologies). Quantitative RT–PCR (qRT–PCR) was used to measure the expression levels of hsp-6 , hsp-60 , timm-23 (primers in Supplementary Table 4 ) and normalization controls pmp-3 and cdc-42 (TaqMan Gene Expression Assays, Life Technologies). The relative standard curve method was used to calculate gene expression. How to cite this article: Bennett, C.F. et al. Activation of the mitochondrial unfolded protein response does not predict longevity in Caenorhabditis elegans . Nat. Commun. 5:3483 doi: 10.1038/ncomms4483 (2014).